Mammalian frataxin directly enhances sulfur transfer of NFS1 persulfide to both ISCU and free thiols Friedreich’s ataxia is a severe neurodegenerative disease caused by the decreased expression of frataxin, a mitochondrial protein that stimulates iron–sulfur (Fe-S) cluster biogenesis. In mammals, the primary steps of Fe-S cluster assembly are performed by the NFS1–ISD11–ISCU complex via the formation of a persulfide intermediate on NFS1. Here we show that frataxin modulates the reactivity of NFS1 persulfide with thiols. We use maleimide-peptide compounds along with mass spectrometry to probe cysteine-persulfide in NFS1 and ISCU. Our data reveal that in the presence of ISCU, frataxin enhances the rate of two similar reactions on NFS1 persulfide: sulfur transfer to ISCU leading to the accumulation of a persulfide on the cysteine C104 of ISCU, and sulfur transfer to small thiols such as DTT, L -cysteine and GSH leading to persulfuration of these thiols and ultimately sulfide release. These data raise important questions on the physiological mechanism of Fe-S cluster assembly and point to a unique function of frataxin as an enhancer of sulfur transfer within the NFS1–ISD11–ISCU complex. Friedreich’s ataxia is a severe neurodegenerative disease caused by the reduced expression of the small globular mitochondrial protein, frataxin (FXN) [1] . In patients and various models of Friedreich’s ataxia, Fe-S cluster biogenesis and iron metabolism are impaired [2] , [3] . Initial studies on eukaryotic and prokaryotic FXNs suggested roles in iron storage [4] , delivery [5] and detoxification [6] , but the physiological relevance of these functions has been questioned [7] , [8] , [9] , [10] . Recent studies instead point to a direct role of FXN in Fe-S cluster assembly [11] , [12] , [13] , [14] . Fe-S clusters are essential prosthetic groups of proteins operating a wide range of functions from enzymatic catalysis, electron transfer to oxidative and nitrosative stress sensing [15] , [16] . In eukaryotes, Fe-S cluster-containing proteins are distributed in almost every cellular compartment, especially in mitochondria, the cytosol and the nucleus [16] . The biogenesis of Fe-S clusters is performed by two main multi-protein machineries, the ISC (Iron–Sulfur Cluster) machinery localized in mitochondria and the CIA (Cytosolic Iron–sulfur cluster Assembly) machinery localized in the cytosol [16] . The ISC machinery provides Fe-S clusters for mitochondrial proteins and also synthesizes an unknown compound that is exported to the cytosol and required for assembly of Fe-S clusters by the CIA machinery [17] , [18] , [19] . The ISC machinery comprises ISCU, a scaffold protein on which Fe-S clusters are assembled, NFS1, a pyridoxal phosphate-dependent cysteine desulfurase, ISD11 and FXN [20] , [21] , [22] , [23] . The eukaryotic ISC machinery has evolved from bacteria and thus some of the primary steps of Fe-S cluster assembly have been conserved [16] , [24] , [25] . As a common strategy, nascent Fe-S clusters are assembled on ISCU from iron and sulfide and transferred to recipient apo-proteins with the assistance of other specialized proteins. The sulfide ions are provided to ISCU in the form of a persulfide intermediate on the catalytic cysteine C383 of NFS1 (NFS1-SSH, where the terminal sulfur is also called sulfane sulfur) by desulfurization of L -cysteine. ISD11 is proposed to stabilize NFS1 and also to promote formation of persulfide on NFS1 (refs 12 , 26 , 27 ). In the bacterial system, the sulfane sulfur of the persulfide carried by IscS, the homologue of NFS1, is transferred to IscU by a trans -persulfuration process leading to poly-persulfurated IscU [28] , [29] , [30] . A similar trans -persulfuration process has been recently decribed with the mammalian system [31] . Unfortunately, mechanistic details of the subsequent steps leading to Fe-S cluster assembly are still lacking. Mammalian FXN was proposed to stimulate the rate of Fe-S cluster assembly by enhancing sulfide production via binding to the NFS1–ISD11–ISCU complex [11] , [14] , [32] . This stimulatory effect was dependent on the presence of ISCU and ultimately favoured the assembly of [4Fe4S] clusters at the expense of [2Fe2S] clusters [11] . In yeast, the homologue of FXN, Yfh1, was proposed to stimulate the formation of persulfide on Nfs1 by increasing the affinity of L -cysteine for Nfs1 (ref. 12 ). Intriguingly, and in stark contrast to the mammalian system, this effect of Yfh1 was independent of the presence of ISCU. In bacteria, CyaY, the homologue of eukaryotic FXN, was shown to slow down rather than stimulate Fe-S assembly on the IscS–IscU complex [33] and did not alter the [2Fe2S]:[4Fe4S] cluster ratio [34] . These contrasting data raise important questions concerning the molecular function of FXN, (both in bacteria and mammals), and the mechanism by which FXN stimulates sulfide production and the rates of Fe-S cluster assembly. To determine the mechanism by which mammalian FXN stimulates Fe-S cluster assembly, we here develop a novel assay to probe protein persulfide that makes use of sulfur-reactive maleimide-peptide compounds. Along with mass spectrometry analysis, the maleimide-peptide assays reveal that the sulfane sulfur of NFS1 is directly and spontaneously transferred to ISCU leading to the accumulation of a persulfide on its cysteine C104. The single-turnover kinetics of formation, reduction and transfer of persulfide, monitored using the maleimide-peptide assay, provide evidence that FXN is not required for persulfide formation on NFS1, but enhances the rate of sulfur transfer to ISCU and cleavage of NFS1 persulfide by external thiols such as L -cysteine and glutathione (GSH), which leads to sulfur transfer on these thiols and ultimately sulfide release. In contrast, FXN does not impact ISCU persulfide reduction. We also show that NFS1 persulfide reduction by thiols is the rate-limiting step in multiple-turnover kinetics and that ISCU persulfide is not reduced under these conditions and thus does not contribute to sulfide release. Thereby, FXN stimulates sulfide release exclusively by enhancing the rate of NFS1 persulfide reduction by thiols. However, this pathway is not efficient for Fe-S cluster assembly on ISCU. These data shed new light on the molecular function of mammalian FXN within the ISC machinery and raise questions on the physiological mechanism of Fe-S cluster assembly. FXN is not required for NFS1 persulfide formation In mammals, the global rate of sulfide production is enhanced by FXN and decreased by ISCU when thiols are used as reductants [11] , [14] , but a step-by-step characterization of the effects of FXN and ISCU on the catalytic cycle of NFS1 is still lacking ( Fig. 1a ). To monitor the formation and reduction of NFS1 persulfide independently, we developed a new assay enabling the detection and quantification of persulfide. This assay is based on the chemical properties of the persulfide group, which contains both a terminal sulfur amenable to alkylation by maleimide compounds and a disulfide bond that can be cleaved by reduction ( Fig. 1b ). In brief, a persulfide is revealed by the loss of the succinimide-peptide moiety (the product of maleimide reaction with a sulfhydryl) upon cleavage of the sulfur–sulfur bond by dithiothreitol (DTT). To visualize the loss of the succinimide moiety, we engineered maleimide compounds with a peptide arm (maleimide-peptide, MalP) of a size sufficiently large to be detected by SDS–polyacrylamide gel electrophoresis (PAGE). The best results were obtained with a 16-mer MalP (MalP 16 : 1.95 kDa) ( Fig. 1c ). In the absence of L -cysteine (the substrate of NFS1), the seven cysteines of NFS1 were alkylated by MalP 16 (denoted NFS1+7 species) and no loss of the succinimide-peptide moiety was observed upon reduction by DTT, indicating that none of NFS1 cysteines was initially persulfurated ( Fig. 1d and Supplementary Fig. 1a ). Following reaction with L -cysteine, the seven cysteines of NFS1 were still alkylated by MalP 16 but reduction by DTT led to the loss of one succinimide-peptide moiety from the NFS1+7 species leading to formation of an NFS1+6 species, thereby indicating the presence of a persulfide group on a single cysteine of NFS1 ( Fig. 1d ). 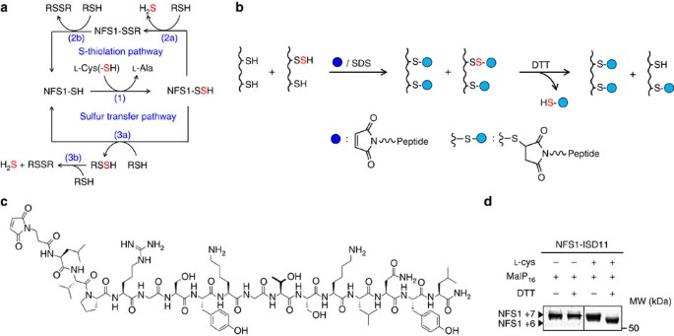Figure 1: Maleimide-peptide assay principle. (a) Catalytic cycle of the cysteine desulfurase NFS1. (1) formation of persulfide on NFS1 (NFS1-SSH) through PLP-catalyzed desulfurization ofL-cysteine that generatesL-alanine as a by-product. NFS1 persulfide can be reduced by thiols (RSH) by two different mechanisms:S-thiolation (2) or sulfur transfer (3). TheS-thiolation pathway leads first to sulfide release andS-thiolation of NFS1 (NFS1-SSR) (2a) and then reduction of NFS1-SSR by a second thiol (2b). The sulfur transfer pathway leads first to sulfur transfer on the thiol that generates a persulfurated thiol (RSSH) (3a) and then hydrogen sulfide after reduction by a second thiol (3b). (b) Reaction scheme of alkylation assay principle by maleimide-peptide (MalP) for identification of persulfide. The reactions of formation and reduction of persulfide are quenched by adding MalP (dark blue) under denaturing conditions (SDS) that alkylates all the thiol groups including persulfurated and non-persulfurated cysteines. The presence of a persulfurated cysteine is revealed by the loss of the succinimide-peptide moiety (light blue) on reduction of the disulfide bond of the persulfide by DTT. The different species are then separated by SDS–PAGE. (c) Structure of the MalP16maleimide-peptide. (d) Maleimide-peptide assay of NFS1 persulfide before and after reaction withL-cysteine. The alkylated forms of NFS1 are indicated as NFS1+7 and NFS1+6 corresponding to seven and six cysteine residues alkylated by MalP16, respectively. Figure 1: Maleimide-peptide assay principle. ( a ) Catalytic cycle of the cysteine desulfurase NFS1. (1) formation of persulfide on NFS1 (NFS1-SSH) through PLP-catalyzed desulfurization of L -cysteine that generates L -alanine as a by-product. NFS1 persulfide can be reduced by thiols (RSH) by two different mechanisms: S -thiolation (2) or sulfur transfer (3). The S -thiolation pathway leads first to sulfide release and S -thiolation of NFS1 (NFS1-SSR) (2a) and then reduction of NFS1-SSR by a second thiol (2b). The sulfur transfer pathway leads first to sulfur transfer on the thiol that generates a persulfurated thiol (RSSH) (3a) and then hydrogen sulfide after reduction by a second thiol (3b). ( b ) Reaction scheme of alkylation assay principle by maleimide-peptide (MalP) for identification of persulfide. The reactions of formation and reduction of persulfide are quenched by adding MalP (dark blue) under denaturing conditions (SDS) that alkylates all the thiol groups including persulfurated and non-persulfurated cysteines. The presence of a persulfurated cysteine is revealed by the loss of the succinimide-peptide moiety (light blue) on reduction of the disulfide bond of the persulfide by DTT. The different species are then separated by SDS–PAGE. ( c ) Structure of the MalP 16 maleimide-peptide. ( d ) Maleimide-peptide assay of NFS1 persulfide before and after reaction with L -cysteine. The alkylated forms of NFS1 are indicated as NFS1+7 and NFS1+6 corresponding to seven and six cysteine residues alkylated by MalP 16 , respectively. Full size image In a first set of experiments, we monitored the influences of ISCU (U) and FXN (F) on the rates of persulfide formation (reaction 1, Fig. 1a ) by the NFS1–ISD11 complex (NI). The NFS1–ISD11 complex (NI), ISCU (U) and FXN (F) have been shown to form homodimeric ternary and quaternary complexes with NI:U and NI:U:F stoichiometries of 1:1 and 1:1:1 for each subunit, respectively [11] , [14] , [23] , which will be denoted NIU and NIUF thereafter. We confirmed here by size exclusion chromatography that when incubated together, these proteins form the NIU and NIUF complex and that FXN does no interact with the NI complex in the absence of ISCU ( Supplementary Fig. 2a–e ). However, by using 100 μM of the NI complex and five equivalents of FXN, only a small proportion of FXN was detected as an NIUF complex, which questioned the efficiency of complex formation at these concentrations. To determine the optimal protein concentration for NIU and NIUF complexes formation, we titrated the amount of FXN and ISCU that would generate the maximal effect on NFS1 cysteine desulfurase activity ( Supplementary Fig. 2f–h ). Maximal attenuation was obtained with 1 molar equivalent of ISCU for 20 μM of the NI complex. In the absence of ISCU, FXN did not alter NFS1 cysteine desulfurase activity, in agreement with the lack of interaction between FXN and the NI complex. In the presence of one equivalent of ISCU, one equivalent of FXN gave the maximal stimulatory effect with 20 μM of the NI complex. At these concentrations, these proteins are thus predominantly in the form of the NIU and NIUF complexes. Moreover, these results are consistent with the reported stoichiometries in the NIU and NIUF complexes [11] . We concluded that the low amount of the NIUF complex detected by size exclusion chromatography at 100 μM was probably due to dissociation of FXN from the NIU complex during elution on the gel filtration column. Under these conditions, NFS1 was almost entirely converted to its persulfurated form (~95%) 10 s after reaction with L -cysteine, and this irrespective of the presence of FXN and/or ISCU ( Fig. 2a ). Mammalian FXN is thus not required for persulfide formation on NFS1, in contrast to what was shown for the yeast homologue of FXN, Yfh1, even when using the concentrations of enzyme and L -cysteine reported in this study ( Supplementary Fig. 1b ) [12] . 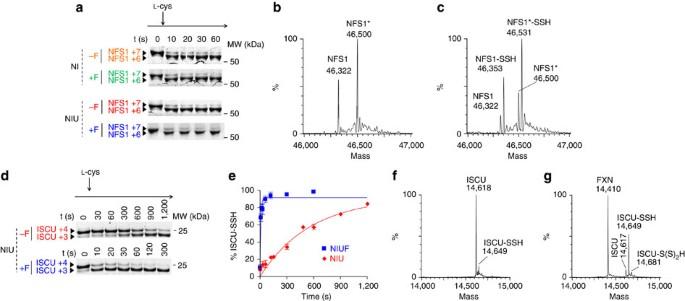Figure 2: Influence of FXN on NFS1 and ISCU persulfide formation. (a) Kinetics of persulfide formation on NFS1 in mixtures containing the NI complex alone (25 μM) or the NI complex (25 μM) and equimolar amounts of ISCU and/or FXN, monitored by alkylation assay. The reaction was initiated by addingL-cysteine and analysed under reducing conditions by SDS–PAGE. The +7 and +6 species represent NFS1 with seven and six cysteines alkylated by MalP16, respectively. (b,c) ESI-Q/TOF spectra of the NI complex before (b) and after (c) reaction withL-cysteine. The asterisk representsN-gluconoylated NFS1. (d) Kinetics of ISCU persulfide formation in the NIU and NIUF complexes (25 μM) monitored by alkylation assay. The reaction is initiated byL-cysteine (500 μM) and analysed under reducing conditions. The different alkylated forms of ISCU are indicated as ISCU+4 and ISCU+3 corresponding to four and three cysteines alkylated by MalP16, respectively. (e) Graphical representation of ISCU persulfide (ISCU-SSH) formation kinetics in the NIU and NIUF complexes determined by quantification of the gels inc. The percentage of ISCU-SSH is defined by the amount of the +3 species relative to the sum (+4+ +3). The solid line represents the best fit using a first-order rate equation. (f,g) ESI-Q/TOF mass spectra of the NIU complex on reaction withL-cysteine in the absence (f) and presence (g) of FXN. The spectra represent a zoom on the 14,000–15,000 range. Figure 2: Influence of FXN on NFS1 and ISCU persulfide formation. ( a ) Kinetics of persulfide formation on NFS1 in mixtures containing the NI complex alone (25 μM) or the NI complex (25 μM) and equimolar amounts of ISCU and/or FXN, monitored by alkylation assay. The reaction was initiated by adding L -cysteine and analysed under reducing conditions by SDS–PAGE. The +7 and +6 species represent NFS1 with seven and six cysteines alkylated by MalP 16 , respectively. ( b , c ) ESI-Q/TOF spectra of the NI complex before ( b ) and after ( c ) reaction with L -cysteine. The asterisk represents N -gluconoylated NFS1. ( d ) Kinetics of ISCU persulfide formation in the NIU and NIUF complexes (25 μM) monitored by alkylation assay. The reaction is initiated by L -cysteine (500 μM) and analysed under reducing conditions. The different alkylated forms of ISCU are indicated as ISCU+4 and ISCU+3 corresponding to four and three cysteines alkylated by MalP 16 , respectively. ( e ) Graphical representation of ISCU persulfide (ISCU-SSH) formation kinetics in the NIU and NIUF complexes determined by quantification of the gels in c . The percentage of ISCU-SSH is defined by the amount of the +3 species relative to the sum (+4+ +3). The solid line represents the best fit using a first-order rate equation. ( f , g ) ESI-Q/TOF mass spectra of the NIU complex on reaction with L -cysteine in the absence ( f ) and presence ( g ) of FXN. The spectra represent a zoom on the 14,000–15,000 range. Full size image We next characterized the persulfide formed on NFS1 by mass spectrometry. The mass spectrum of NFS1 displayed two peaks, one at 46,322±1 Da, identified as NFS1 (expected mass of 46,322 Da) and the other one at 46,500±1 Da ( Fig. 2b ), attributed to an N -gluconoylated form of NFS1 (+178 Da) either on the first histidine of the His-tag or on the NH 2 N-terminus of NFS1 (ref. 35 ), as shown by LC-ESI-ORBITRAP-MS/MS characterization of the peptide mass fingerprint ( Supplementary Fig. 3a,b and Supplementary Table 1 ). Upon reaction of the NI complex with L -cysteine, two major species were detected, corresponding to NFS1 and its N -gluconoylated form each carrying a mass increment of 32±1 Da, consistent with the incorporation of a single sulfur atom ( Fig. 2c ). About 30% of non-persulfurated NFS1 was also detected that probably originates from the loss of the sulfane sulfur under the conditions of mass spectrometry [36] , as this species was not detected by the alkylation assay. Similar species were detected when the NI complex was reacted with L -cysteine in the presence of FXN and/or ISCU ( Supplementary Fig. 3c–e ). These results establish that the main species characterized by the maleimide-peptide assay are mono-persulfurated forms of NFS1. Importantly, these data confirm the results of the maleimide-peptide assay indicating that FXN is not required for persulfide formation on NFS1. FXN enhances sulfur transfer from NFS1 persulfide to ISCU We next investigated persulfide transfer from NFS1 to ISCU using the maleimide-peptide assay ( Fig. 2d ). Before reaction of the NIU complex with L -cysteine and upon reaction with MalP 16 , the majority of ISCU carried four succinimide-peptide moieties (denoted ISCU+4, see Supplementary Fig. 1c ). A small amount of ISCU (<5%) was mono-persulfurated (ISCU+3) as a result of persulfuration of the overexpressed protein within bacteria. Residual amounts of this persulfurated form were still present after reduction by DTT (see Methods). On reaction of the NIU complex with L -cysteine, the ISCU+4 species was gradually converted to the ISCU+3 species ( Fig. 2d,e ). Remarkably, when the reaction was performed in the presence of FXN, the conversion occurred about 50-fold faster ( Table 1 ). These results indicate that FXN enhances the rate of persulfide formation on ISCU. Table 1 Effects of FXN and ISCU on the single turnover kinetic parameters. Full size table Mass spectrometry analysis showed that after 3 min of reaction of the NIU complex with L -cysteine, ISCU was detected as a main peak at 14,618±1 Da that closely matched the theoretical mass of reduced ISCU (expected mass 14,618 Da) and as a minor peak at 14,649±1 Da that corresponds to a mono-persulfurated form of ISCU (expected mass of 14,650 Da) ( Fig. 2f and Supplementary Fig. 3f ). When the reaction was performed in the presence of FXN, ISCU was almost entirely converted into the mono-persulfurated form with a minor fraction present as a bis-persulfurated form (expected mass of 14,682 Da; Fig. 2g and Supplementary Fig. 3g ). These data confirm that, as observed with the maleimide-peptide assay, FXN enhances sulfur transfer to ISCU, and also establish that the species persulfurated on a single cysteine are mainly mono-persulfurated forms of ISCU. To establish which of the four cysteine residues of ISCU is(are) modified, tryptic digests of the NIU and NIUF complexes were analysed by LC-ESI-ORBITRAP-MS/MS followed by MS/MS ( Table 2 , Supplementary Fig. 4a–d and Supplementary Table 2 ). All four ISCU cysteine-containing peptides were detected, and only those containing C35 and C104 were detected with a persulfide, both in the NIU and NIUF complexes. Semi-quantitative analysis indicated that C104 was persulfurated by 65% in the NIU complex and by 60% in the NIUF complex, whereas C35 was persulfurated by 2–5% in either complex ( Table 2 ). To assess which ISCU cysteine is the primary persulfide receptor, we prepared cysteine-to-serine substitution mutants of the three conserved ISCU cysteines C35, C61 and C104 (C35S, C61S and C104S mutants) and used them in the reaction system. The C61S mutant was only expressed as a truncated polypeptide that did not inteact with the NI complex and was therefore discarded ( Supplementary Fig. 5 ). The C35S and C104S ISCU mutants were expressed as full-length polypeptides that could form a ternary complex with the NI complex. Using the maleimide-peptide assay, we observed that the persulfuration of ISCU was abolished with both the C104S and C35S mutants, and was not influenced by FXN ( Fig. 3 ). These data indicate that C35 and C104 are both important for trans -persulfuration and/or that each of these mutations alter the trans -persulfuration process potentially by modifying the structure of the putative Fe-S cluster-binding site. Although these data cannot tell which of C35 or C104 is the primary ISCU receptor of NFS1 persulfide, they clearly establish that C104 is the major sink of persulfide on ISCU. Table 2 Identification of ISCU persulfurated peptides in the NIU and NIUF complex. 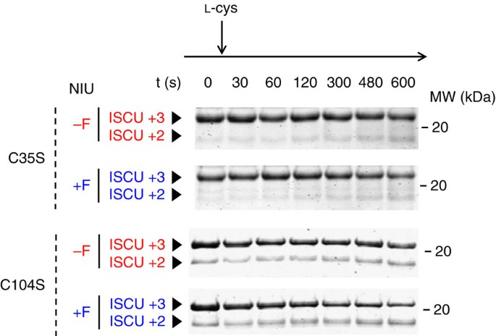Figure 3: Identification of the persulfurated cysteines of ISCU. Alkylation assays with C35S and C104S ISCU mutants. The kinetics of ISCU persulfide formation in the NIU and NIUF complexes (25 μM) prepared with the C35S and C104S ISCU mutants were initiated withL-cysteine (500 μM) and analysed under reducing conditions. The +3 and +2 species represent non-persulfurated and persulfurated ISCU mutants, respectively. Full size table Figure 3: Identification of the persulfurated cysteines of ISCU. Alkylation assays with C35S and C104S ISCU mutants. The kinetics of ISCU persulfide formation in the NIU and NIUF complexes (25 μM) prepared with the C35S and C104S ISCU mutants were initiated with L -cysteine (500 μM) and analysed under reducing conditions. The +3 and +2 species represent non-persulfurated and persulfurated ISCU mutants, respectively. Full size image We then enquired how the persulfide is transferred from NFS1 to ISCU, whether directly from the PLP cofactor of NFS1, from NFS1 persulfide or via small thiol-containing carriers, specifically L -cysteine. Persulfurated NFS1 (NFS1-SSH) was first generated, excess L -cysteine was then removed and ISCU alone or together with FXN were added. We observed that concomitant to the disappearance of NFS1 persulfide, ISCU became persulfurated. Moreover, the rate of ISCU persulfuration measured in the absence of L -cysteine was similar to the one measured in its presence ( Supplementary Fig. 6a,b ). These data indicate that the transfer of sulfur proceeds by a direct attack of one of ISCU cysteine on NFS1 persulfide in both the NIU and NIUF complexes. So far we have shown that FXN is not required for persulfide formation on NFS1 but stimulates sulfur transfer from NFS1 persulfide to ISCU which could explain the stimulatory effect of FXN on the global rate of sulfide production, if ISCU persulfide is reduced faster than NFS1 persulfide and is thus the main source of sulfide. To assess this hypothesis, we sought to determine the individual rates of persulfide reduction for NFS1 and ISCU and to investigate the influence of FXN on the rates of these reactions. FXN enhances sulfur transfer from NFS1 persulfide to DTT We first investigated the reaction of NFS1 persulfide reduction with DTT. The persulfides were generated on NFS1 and ISCU by incubating mixtures of equimolar amounts of NFS1–ISD11, ISCU and FXN with L -cysteine. Then, L -cysteine was removed, as it would regenerate the persulfide on NFS1 following its reduction, and DTT was added. We first noticed that NFS1 persulfide reduction was much slower than its formation ( Fig. 4a , and see Fig. 2a ), which indicated that reduction of NFS1 persulfide is the rate-limiting step of the cysteine desulfurase cycle under these conditions (reaction 2 or 3, Fig. 1a ). Remarkably, ISCU and FXN both altered the rate of NFS1 persulfide reduction, but in opposite ways ( Fig. 4a,b ). While the binding of ISCU to the NI complex slowed down the reaction, the binding of FXN to the NIU complex enhanced it, but had no effect on the NI complex. The data were fitted assuming that reduction of NFS1 persulfide by DTT is a bimolecular reaction (see below, see also Methods; Table 1 ). The values of the rate constants indicated that ISCU slows down the reaction by fivefold and FXN stimulates the reduction of NFS1 persulfide by approximately 25-fold as compared with NIU. 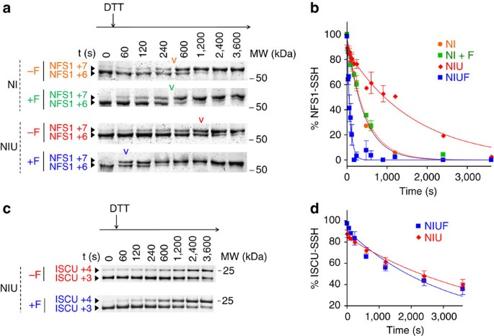Figure 4: Influence of FXN on the reduction of NFS1 and ISCU persulfides. (a) Kinetics of NFS1 persulfide reduction in mixtures containing the NI complex alone (25 μM) or the NI complex (25 μM) and equimolar amounts of ISCU and/or FXN, monitored by alkylation assay. The reaction was initiated by DTT (1 mM) and analysed under reducing conditions. The reduction of NFS1 persulfide was characterized by appearance of the NFS1+7 species. The ‘v’ symbol indicates the time to reach 50% reduced NFS1. (b) Graphical representation of NFS1 persulfide reduction kinetics determined from quantification of the gels ina. The percentage of NFS1-SSH is defined by the amount of the +6 species relative to the sum (+7 + +6). The solid line represents the best fit using a second-order rate equation. (c) Kinetics of ISCU persulfide reduction in the NIU and NIUF complexes (25 μM) monitored by alkylation assay. The reaction is initiated with DTT (1 mM) and analysed under reducing conditions. The reduction of ISCU-SSH is characterized by the appearance of the +4 species corresponding to non-persulfurated ISCU. (d) Graphical representation of ISCU persulfide (ISCU-SSH) reduction kinetics in the NIU and NIUF complexes, determined by quantification of the gels inc. The solid line represents the best fit using a second-order rate equation. Figure 4: Influence of FXN on the reduction of NFS1 and ISCU persulfides. ( a ) Kinetics of NFS1 persulfide reduction in mixtures containing the NI complex alone (25 μM) or the NI complex (25 μM) and equimolar amounts of ISCU and/or FXN, monitored by alkylation assay. The reaction was initiated by DTT (1 mM) and analysed under reducing conditions. The reduction of NFS1 persulfide was characterized by appearance of the NFS1+7 species. The ‘v’ symbol indicates the time to reach 50% reduced NFS1. ( b ) Graphical representation of NFS1 persulfide reduction kinetics determined from quantification of the gels in a . The percentage of NFS1-SSH is defined by the amount of the +6 species relative to the sum (+7 + +6). The solid line represents the best fit using a second-order rate equation. ( c ) Kinetics of ISCU persulfide reduction in the NIU and NIUF complexes (25 μM) monitored by alkylation assay. The reaction is initiated with DTT (1 mM) and analysed under reducing conditions. The reduction of ISCU-SSH is characterized by the appearance of the +4 species corresponding to non-persulfurated ISCU. ( d ) Graphical representation of ISCU persulfide (ISCU-SSH) reduction kinetics in the NIU and NIUF complexes, determined by quantification of the gels in c . The solid line represents the best fit using a second-order rate equation. Full size image Two different mechanisms of reduction by thiols are feasible, through S -thiolation of NFS1 or sulfur transfer to the thiol ( Fig. 1a ). In the case of the S -thiolation pathway, a DTT adduct is expected that will appear as an NFS1+6 species under non-reducing conditions in the alkylation assays. Under these conditions, no NFS1+6 species was detected ( Supplementary Fig. 6c ), indicating that NFS1 persulfide is reduced through sulfur transfer on DTT. We thus conclude that FXN stimulates and ISCU slows down sulfur transfer to DTT and that the effect of FXN relies on the presence of ISCU. FXN does not enhance ISCU persulfide reduction We next examined the influence of FXN on the rate of ISCU persulfide reduction by DTT starting from fully persulfurated forms of both NFS1 and ISCU. The rates of ISCU persulfide reduction were similar in the absence or presence of FXN ( Fig. 4c,d ), indicating that FXN does not affect this step. The comparison of the respective rate constants of ISCU and NFS1 persulfide reduction by DTT indicated that reduction of NFS1 persulfide is faster than reduction of ISCU persulfide, by threefold in the absence of FXN and 45-fold in its presence ( Table 1 ), suggesting that ISCU may not contribute to the global sulfide production when DTT is used as a reductant. Taken together, the results of the single-turnover kinetics indicate that FXN enhances the rate of two reactions: sulfur transfer to ISCU and sulfur transfer to DTT. However, since DTT is not a physiological reductant, we wondered whether the effect of FXN and the differences in the rates of persulfide reduction between NFS1 and ISCU could be observed with physiologically relevant reductants. L -cysteine and GSH reduce NFS1 persulfide Using the maleimide-peptide assay, we assayed persulfide reductase activities of two electron donors postulated to enable persulfide reduction [37] , [38] , [39] , ferrous iron (Fe 2+ ) and mammalian mitochondrial ferredoxin 2, FDX2, in its reduced state. Neither iron alone or together with FDX2 had an impact on NFS1 or ISCU persulfides ( Supplementary Fig. 7a ). We thus tested the thiol-containing molecules, GSH, which contributes to cytosolic Fe-S cluster assembly in yeast by a still undefined mechanism [40] , [41] and L -cysteine. GSH did not affect ISCU persulfide even after 60 min, but could reduce NFS1 persulfide ( Supplementary Fig. 7b ) albeit at a rate approximately 140-times lower than DTT ( Table 1 ). To test L -cysteine, the maleimide-peptide assay could not be used since L -cysteine would regenerate NFS1 persulfide following its reduction. We instead monitored L -alanine production ( Fig. 5a ). For each concentration of L -cysteine, the amount of L -alanine generated exceeded the concentration of the NI complex, which indicated that several turnovers were achieved and thus that L -cysteine was able to reduce NFS1 persulfide. Cystine (oxidized cysteine), which is the expected by-product of persulfide reduction by L -cysteine, was concomitantly generated in the reaction mixture, further supporting this conclusion ( Supplementary Fig. 7c–e ). To determine whether L -cysteine reduces NFS1 through sulfur transfer or S -thiolation ( Fig. 1a ), we analysed the kinetics of persulfide formation under non-reducing conditions since an NFS1+6 species is expected to appear in the case of the S -thiolation pathway. No L -cysteine adduct was detected under these conditions, which is consistent with the sulfur transfer mechanism of reduction ( Fig. 1d and Supplementary Fig. 1b ). Moreover, the kinetics of Fe-S cluster reconstitution performed with L -cysteine as a reductant (without DTT), displayed a lag phase indicative of a delay in sulfide release ( Supplementary Fig. 8a–c ). Such a lag phase is not expected in the case of the S -thiolation mechanism for which sulfide release should initiate immediately upon adding L -cysteine, whereas it is consistent with the sulfur transfer mechanism for which sulfide release is not directly correlated with NFS1 persulfide reduction but with the subsequent step of reduction of the persulfurated thiol ( Fig. 1a , reaction (3b)). These data thus further support the sulfur transfer mechanism. 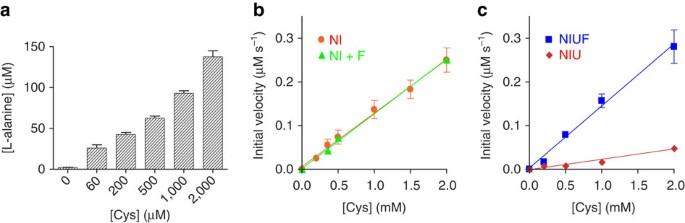Figure 5: Effects of FXN on the NFS1–ISD11–ISCU complex in multiple-turnover kinetics. (a) Effects ofL-cysteine concentration on the amount ofL-alanine produced by the NIUF complex. The reactions were performed with the NIUF complex (20 μM) and increasing amounts ofL-cysteine in the absence of DTT.L-alanine production was monitored by ADH assays after 10 min of reaction. (b,c) Effect of FXN and ISCU on the initial velocities ofL-alanine formation under steady-state conditions. The NI complex (20 μM) alone and with equimolar amounts of FXN (b) and the NIU and NIUF complexes (20 μM) (c) were incubated with various amounts ofL-cysteine and the initial velocities were plotted as a function ofL-cysteine concentrations. The bars represent the s.e. from three independent experiments. The lines represent the linear regression. Figure 5: Effects of FXN on the NFS1–ISD11–ISCU complex in multiple-turnover kinetics. ( a ) Effects of L -cysteine concentration on the amount of L -alanine produced by the NIUF complex. The reactions were performed with the NIUF complex (20 μM) and increasing amounts of L -cysteine in the absence of DTT. L -alanine production was monitored by ADH assays after 10 min of reaction. ( b , c ) Effect of FXN and ISCU on the initial velocities of L -alanine formation under steady-state conditions. The NI complex (20 μM) alone and with equimolar amounts of FXN ( b ) and the NIU and NIUF complexes (20 μM) ( c ) were incubated with various amounts of L -cysteine and the initial velocities were plotted as a function of L -cysteine concentrations. The bars represent the s.e. from three independent experiments. The lines represent the linear regression. Full size image Altogether, the single-turnover kinetics indicate that thiols such as DTT, L -cysteine and GSH are able to reduce NFS1 and ISCU persulfides but these reactions are not synchronized. The reduction of NFS1 persulfide by thiols is apparently more efficient than the reduction of ISCU persulfide. We have thus asked whether the reduction of ISCU contributes to sulfide release in multiple-turnover kinetics. Thiol-dependent sulfide release is mediated by NFS1 persulfide We investigated the influence of FXN on the rate of L -alanine production. Analysis of multiple-turnover kinetics under steady-state conditions is also a powerful tool to determine the mechanism by which L -cysteine reduces protein persulfide. Two mechanisms were considered: (i) formation of an enzyme–substrate complex as described by the Michaelis–Menten model for which the initial velocity reaches a plateau when the concentration of substrate increases as the enzyme becomes saturated [42] and (ii) a bimolecular process for which non-saturation behaviour is expected. We thus measured initial velocities of L -alanine production under steady-state conditions (see Methods) for various concentrations of L -cysteine. The variations of the initial velocities of L -alanine formation by the NI complex alone or in the presence of equimolar amounts of FXN and/or ISCU displayed a linear relationship with the concentration of L -cysteine up to 2 mM ( Fig. 5b,c ). Such behaviour is a feature of bimolecular reactions. A similar mechanism was reported for the IscS-like cysteine desulfurase Slr0387 from Synechocystis sp. PCC 6803 that exhibited second-order kinetic with thiols as reducers of the persulfide [43] . However, saturation behaviours that were interpreted using the Michaelis–Menten model, were obtained by other groups with mammalian NFS1 using higher L -cysteine to NFS1 ratios (1,000 equivalents of L -cysteine for the highest concentration versus 100 equivalents of L -cysteine here) [11] , [14] , [32] . By increasing L -cysteine concentration above 2 mM, we indeed observed that the variation of the initial velocity deviated from linearity and even decreased at very high L -cysteine concentrations for the NIU complex ( Supplementary Fig. 9a ). Analysis using the Michaelis–Menten equation yielded K M values in the range of 50–150 mM. These K M values are unlikely physiological. Moreover, they are much higher than those reported earlier, that is, in the 10–40 μM range [11] , [14] , [32] , indicating that the K M values are concentration dependent, which is not consistent with an enzyme–substrate model. L -cysteine and DTT were reported to inhibit the cysteine desulfurase Slr0387 from Synechocystis sp. PCC 6803 and NifS from E. coli [43] , [44] . Therefore, we hypothesized that the saturation behaviours observed by other groups with NFS1 could be due to inhibition caused by L -cysteine itself at ratios above 100 equivalents. The bimolecular rate constants determined by linear regression of the data indicated that FXN did not alter the rate of L -alanine production by the NI complex but significantly enhanced it in the presence of ISCU ( Fig. 5b,c and Table 3 ). Conversely, the binding of ISCU to the NI complex decreased the rate of L -alanine production by the NI complex. These effects are reminiscent of the effects of FXN and ISCU on NFS1 persulfide reduction by DTT observed by single-turnover kinetics (see Fig. 4a,b ). However, in these multiple-turnover kinetics, the reduction of ISCU persulfide may also contribute to the global rate of L -alanine production, we thus sought to determine the rate-limiting step of the catalytic cycle. Table 3 Effects of FXN and ISCU on the multiple turnover kinetic parameters. Full size table To selectively disturb persulfide reduction without affecting its formation, we examined the influence of DTT on the global rate of L -alanine production, since DTT is only involved in the reduction step. We observed that the initial velocity of L -alanine production increased with the concentration of DTT, which is a first indication that reduction is rate-limiting ( Supplementary Fig. 9b ). This conclusion was supported by a second observation. The plot of L -alanine formation by the NI complex alone or in the presence of FXN and/or ISCU, when extrapolated to t =0 did not intersect the y axis at y =0 and the amount of L -alanine generated was correlated to the amount of complex ( Supplementary Fig. 9c–g ). This initial burst represents the amount of L -alanine generated during the first half-turnover of NFS1 persulfide formation (reaction 1, Fig. 1a ) and the following part of the reaction ( t >0) reflects subsequent turnovers for which reduction is now required. The respective rates of these two different phases:>20 μM s −1 for persulfide formation and in the range of 0.1 to 1 μM s −1 for the second part indicate that reduction is slowing down the reaction and thus that it is the rate-limiting step. A similar initial burst was observed in the absence of DTT with L -cysteine as the reductant, indicating that reduction is still rate limiting under this condition ( Supplementary Fig. 9h ). The single-turnover kinetics indicated that the reduction of ISCU persulfide by thiols is slower than the reduction of NFS1 persulfide and we confirmed that ISCU persulfide does not contribute to the global rate of L -alanine production by measuring the rates of L -alanine production by the NIU complexes assembled from the C104S and C104G ISCU mutants that are non-persulfurable ( Supplementary Fig. 9i ). Moreover, the bimolecular rate constants for reduction by DTT determined from the multiple turnover experiments were in very good agreement with those determined in single turnover for reduction of NFS1 persulfide by DTT (compare Tables 1 and 3 for DTT). We thus identify persulfide reduction as the rate-limiting step of the catalytic cycle, while ISCU persulfide reduction does not contribute. These results establish that FXN stimulates and ISCU slows down the reduction of NFS1 persulfide by thiols. The functional role of the small mitochondrial protein FXN has been the focus of much interest since its discovery [8] . Only recently it was demonstrated that FXN associates with the early components of the mitochondrial Fe-S cluster biogenesis pathway, NFS1 and ISCU [2] , [23] . It was then reported that in the presence of ISCU, mammalian FXN stimulates sulfide production by NFS1 and this was correlated with stimulation of Fe-S cluster assembly [11] , [14] . Here we confirm that FXN interacts with the ternary NFS1–ISD11–ISCU (NIU) complex to form a quaternary NFS1–ISD11–ISCU–FXN (NIUF) complex. Our titration assays indicate that FXN is mainly associated with the NIU complex at 20 μM and similar results were obtained by other groups with protein concentrations down to 1 μM [11] , [14] , which means that the dissociation constant of the NIUF complex is much lower than 1 μM. However, the size exclusion chromatography profiles show that FXN dissociates from the NIU complex during elution at 100 μM, whereas ISCU remained associated with NFS1 in the same conditions. These observations suggest that the inteaction of FXN with the NIU complex may be more dynamic than the interaction of ISCU with NFS1 (rapid versus slow dissociation) as also proposed in another study [45] and possibly to facilitate exchange with other accessory proteins on the NIU complex. We have then studied the mechanism by which FXN may stimulate Fe-S cluster assembly. Here we show that FXN modulates the rate of sulfur transfer to ISCU and reduction of NFS1 persulfide by free thiols. To reach this conclusion, we have developed a novel method to probe and quantify protein persulfides. This assay is based on detection of protein gel mobility shifts upon reduction of persulfurated cysteine labelled with synthetic maleimide-peptide and was validated by direct identification of persulfide through mass spectrometry analysis. Compared with the other techniques described for identification of persulfide [46] , [47] , [48] , the peptide-maleimide assay provides additional advantages, including the small number of steps required before analysis, its selectivity and owing to its ratiometric nature it provides an accurate quantification of the ratio of persulfurated versus non-persulfurated species. Moreover, it is the first assay enabling determination of the number of persulfurated cysteine residues. This assay was a powerful tool to disentangle formation, reduction and transfer of NFS1 persulfide and thereby to study single-turnover kinetics of these reactions. We have characterized the different events triggered by the reaction of NFS1 with L -cysteine and we have estimated the rates of the these reactions. The reaction is initiated by the formation of a persulfide on NFS1, which is the fastest reaction of the catalytic cycle. The sulfane sulfur of NFS1 persulfide is then rapidly transferred to ISCU in a trans -persulfuration process leading to persulfuration of ISCU on one of its cysteine residues. Upon regeneration of NFS1 persulfide by L -cysteine, this persulfide is reduced by external thiols such as DTT, GSH and L -cysteine. The reduction of NFS1 persulfide likely proceeds by sulfur transfer rather than S -thiolation ( Fig. 1a ). ISCU persulfide is also reduced by external thiols but at a markedly slower rate than NFS1 persulfide. The analysis by mass spectrometry indicates that the persulfides generated on NFS1 and ISCU are mainly mono-persulfides. Although we cannot firmly establish which of the three conserved cysteine of ISCU (C35, C61 or C104) is the primary receptor of NFS1 persulfide, we have identified C104 as the main persulfurated cysteine of ISCU. We have also demonstrated that this reaction is direct and proceeds by a direct nucleophilic attack of one ISCU cysteine on the persulfide of NFS1. We have then investigated the influence of FXN on these reactions. The single-turnover kinetics first provide evidence that formation of NFS1 persulfide reaches ≈95% completion in 10 s, irrespective of the presence of ISCU and/or FXN. We thus conclude that FXN is not required for persulfide formation of NFS1 as confirmed by mass spectrometry analysis. These results challenge two recent studies reporting a stimulatory effect of FXN and its yeast homologue, Yfh1, on NFS1 persulfide formation [12] , [31] . In these studies, the formation of persulfide was monitored using 35 S labelling of L -cysteine. Unfortunately, as the persulfide were not protected by alkylation before running electrophoresis under denaturating conditions, it is not excluded that they were reduced or exchanged with other cysteines, which may explain the discrepancy between our respective studies. However, since the formation of NFS1 persulfide was almost complete in 10 s for all the complexes, we cannot exclude the possibility that FXN stimulates persulfide formation on a timescale below 10 s. The single-turnover kinetics reveal that FXN enhances the rate of sulfur transfer from NFS1 persulfide to ISCU and sulfur transfer of NFS1 persulfide to the small thiol-containing molecule DTT, L -cysteine and GSH. Conversely, ISCU slows down sulfur transfer to these thiols. In contrast, FXN does not alter the rate of ISCU persulfide reduction. The multiple-turnover kinetics indicate that the reduction of NFS1 persulfide is the rate-limting step of the catalytic cycle, hence that the effects of FXN and ISCU on the global rate of the reaction are only related to a modulation of the rate of NFS1 persulfide transfer to these thiols, regardless of a possible additional effect of FXN on NFS1 persulfide formation. These data confirm the results of the single-turnover kinetics. The reduction step is also the rate-limiting reaction of the catalytic cycle of other group I cysteine desulfurases, which suggests that this might be a common feature of this class of enzymes [43] , [44] , [49] . Taken together, our results thus point to a unique molecular function of FXN as an enhancer of sulfur transfer to ISCU and small free thiols ( Fig. 6 ). Sulfide release does occur subsequently, upon condensation of the persulfurated thiol with a second thiol ( Fig. 1a , reaction (3b)), but is not directly catalysed by FXN. 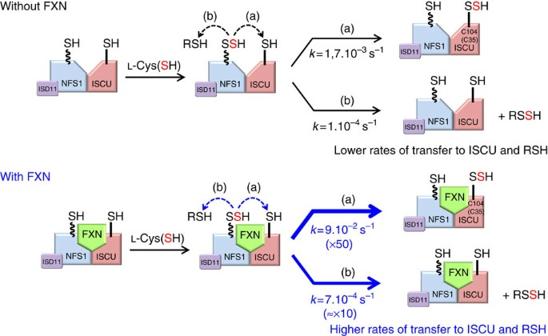Figure 6: Molecular model for the function of FXN in the ISC machinery. In the presence of FXN, the rates of two reactions are enhanced (a) sulfur transfer to ISCU and (b) sulfur transfer to free thiol-containing molecules (RSH) such asL-cysteine and GSH. The rate constants are indicated. For comparison of the rates of transfer to ISCU and RSH, a first-order rate constant for sulfur transfer to RSH has been computed assuming a concentration of 100 μM ofL-cysteine that is close to the physiological concentration50. Figure 6: Molecular model for the function of FXN in the ISC machinery. In the presence of FXN, the rates of two reactions are enhanced (a) sulfur transfer to ISCU and (b) sulfur transfer to free thiol-containing molecules (RSH) such as L -cysteine and GSH. The rate constants are indicated. For comparison of the rates of transfer to ISCU and RSH, a first-order rate constant for sulfur transfer to RSH has been computed assuming a concentration of 100 μM of L -cysteine that is close to the physiological concentration [50] . Full size image These results rule out the hypothesis that FXN stimulates sulfide release by enhancing persulfide formation on NFS1, as proposed by others [11] , [12] , [14] , [31] . FXN has also been proposed to stimulate iron entry within the NIU complex in Fe-S cluster reconstitution assays with DTT [11] . However, since the stimulation of sulfide release, in turn increases the amount of iron bound in the form of Fe-S clusters, the higher proportion of iron bound to the NIUF complex versus the NIU complex, might be a consequence of the enhancement of sulfide production by FXN. These data raise several questions on the physiological mechanism of Fe-S cluster biogenesis: what is the respective role of the two reactions of transfer? Are these reactions correlated with physiologically relevant Fe-S cluster assembly on ISCU? We first determined that ISCU persulfide does not contribute to sulfide release and is not even reduced in Fe-S cluster reconstitution assays when thiols are used as reductants ( Supplementary Fig. 10a–d ). Thus, under these conditions, sulfide production arises exclusively from reduction of NFS1 persulfide and FXN drives Fe-S cluster assembly by enhancing this reaction. However, the rate of Fe-S cluster assembly is slow when DTT and/or L -cysteine are used as reductants (1 h to complete reconstitution on ISCU with L -cysteine) and the reconstitution is inefficient as at least 30 equivalents of sulfide ions are produced in 1 h with L -cysteine (according to the rate constants, Table 3 ) while only two equivalents would be required for building up a [2Fe2S] cluster ( Supplementary Figs 8 and 10 ). These observations suggest that L -cysteine (and also GSH which is an even less efficient reducer of NFS1 persulfide) are not the physiological reductants or that other accessory proteins might be required to secure Fe-S cluster assembly. More likely, since FXN specifically activates sulfur transfer to ISCU, the persulfuration of ISCU might have a functional role in Fe-S cluster assembly but a dedicated reductase is lacking in the Fe-S cluster reconstitution assays. The human ferredoxin FDX2, which provides electrons for Fe-S cluster biogenesis [38] , [39] , is a potential candidate for the reduction of ISCU. However, under our conditions, we were not able to measure any persulfide reductase activity with FDX2. Nervertheless, we cannot exclude that under physiological conditions, FDX2 could be involved in the reduction of ISCU and NFS1 persulfides by a mechanism that still needs to be defined. Following this hypothesis, the stimulation of sulfur transfer to small thiol molecules by FXN may serve another function, possibly sulfur trafficking within the cell. Collectively, our data point to a specific role of FXN in the control of NFS1 persulfide reduction by thiols, enhancing sulfur transfer to both ISCU and free thiols such as L -cysteine and GSH. These data shed new light on the molecular function of FXN and on the early steps of Fe-S cluster assembly by raising important physiological questions on the mechanism of Fe-S cluster biogenesis. Chemicals and biochemical products Luria Bertani medium, protease inhibitor cocktail, N,N' -diisopropylcarbodiimide, DTT, dithionite, trichloroacetic acid (TCA), L -cysteine, L -alanine, L -cystine, L -alanine dehydrogenase (ADH), β-nicotinamide adenine dinucleotide hydrate (NAD + ), ferrous ammonium sulfate (Fe(NH 4 ) 2 (SO 4 ) 2 ), His 6 -thrombin, iodoacetamide (IAA) were from Sigma-Aldrich; isopropyl-β- D -1-thiogalactopyranoside was from AppliChem; disuccinimidyl tartrate from Pierce; trypsin (sequence grade) from Promega; Fmoc-amino acids and the Rink amide p -methylbenzlhydrylamine support were from Novabiochem; 3-maleimidopropanoic acid was from Bachem; 1-hydroxybenzotriazole (HOBt·H 2 O) from Acros Organics and ACCQ-fluo reagent kit from Waters. HiTrap chelating HP column (5 ml), HiPrep Desalting 26/10, HiLoad 26/600 prep grade Superdex 200 and Superdex 75 columns were from GE Healthcare; Amicon Ultra centrifugal filter ultracel 10 and 30 kDa from MILLIPORE, MicroBio-Spin6 columns from Bio-Rad; Rosetta2-(DE3) and pET28b from Novagen. Plasmid and cell culture purification The vectors expressing NFS1-(amino acid (aa) 59 to 459), ISD11, ISCU-(aa 36–168) and FXN-(aa 79–207) were kindly provided by Dr Hélène Puccio (IGBMC, Strasbourg) and their construction was reported earlier [11] . His-tags followed by thrombin (Thr) cleavage sites were introduced by mutagenesis leading to the expression plasmids pCDFDuet-(site1):His 6 -Thr-NFS1-(site2):ISD11, pETDuet-(site1):His 6 -Thr-ISCU and pET16-His 6 -Thr-FXN. The C35S, C61S, C104S and C104G mutations were introduced in ISCU by site-directed mutagenesis (IMAGIF platform, Gif Sur Yvette, France). The vectors expressing human His 6 -Thr-FDX2 (aa 53–183) from pET28b were generated by GenScript (Piscataway, USA). The Rosetta2-(DE3) cells were transformed with the plasmids and the cells were grown from a single colony at 180 r.p.m. at 37 °C in Luria Bertani medium with appropriate antibiotics. Protein expression was induced when the cells reached OD 600 =0.6 using 500 μM isopropyl-β- D -1-thiogalactopyranoside and the cells incubated for an additional 16 h at 18 °C at 180 rpm. The cell cultures were harvested by centrifugation at 5,500 r.p.m. for 10 min at 4 °C. Cell pellets were resuspended in buffer A (50 mM Na 2 HPO 4 , 150 mM NaCl, 5 mM imidazole, pH 8) containing a protease inhibitor cocktail. The cell suspensions were lysed by three cycles of French Press. Cell debris were removed by centrifugation at 45,000 r.p.m. for 45 min at 4 °C. The His-tagged proteins NFS1–ISD11, ISCU (WT and mutants), FXN and FDX2 were purified on a HiTrap chelating HP loaded with nickel ions. The resin was washed with buffer A and bound proteins were eluted by a linear gradient between buffer A and buffer B (50 mM Na 2 HPO 4 , 150 mM NaCl, 500 mM imidazole, pH 8). Protein fractions were mixed and concentrated on Amicon 10 or 30 kDa to 4 ml. The partially purified His 6 -NFS1–ISD11 complex was incubated for 10 min with 10 mM DTT at room temperature to remove persulfide and then loaded on a HiLoad 26/600 Superdex 200 prep grade column pre-equilibrated with buffer C (50 mM Na 2 HPO 4 , 150 mM NaCl, pH 8). The His-tag could not be removed from the NFS1–ISD11 complex as cleavage by thrombin yields non-specific cleavages. The ISCU (WT and mutants), FXN and FDX2 proteins were buffer exchanged on HiPrep Desalting 26/10 and the His-tags were successfully removed by treatment with thrombin (3.5 NIH unit of His 6 -thrombin per mg of proteins) for 16 h at 22 °C. Before thrombin cleavage, ISCU and FXN both migrate as a double band on SDS–PAGE, indicating that significant amounts of these proteins were partially modified. We have attributed this modification to an N -gluconoylation of the His-tag as described for NFS1 ( Fig. 2b,c , Supplementary Fig. 3a,b and Supplementary Table 1 ), since FXN and ISCU are no longer modified after cleavage of the His-tag according to mass spectrometry ( Fig. 2f,g ). The His-tag fragments and His 6 -thrombin were removed by purification on a HiTrap chelating HP loaded with nickel ions and equilibrated with buffer A. The ISCU proteins (WT and mutants) were incubated with 10 mM DTT for 10 min to remove persulfide. The ISCU (WT and mutants) and FDX2 proteins were loaded on a HiLoad 26/600 Superdex 75 prep grade column pre-equilibrated with buffer C. All the proteins were aliquoted and stored in glycerol (10% final) at −80 °C. Protein concentrations were determined from absorbance at 280 nm. The purified C61S ISCU mutant migrated on SDS–PAGE with an apparent molecular weight of 10 kDa suggesting that the protein is truncated. Formation of complexes by size exclusion chromatography The formation of complexes was analysed by size exclusion chromatography using a Superdex S200 10/300 column (GE Healthcare). The proteins were mixed together in buffer C and eluted at a flow rate of 0.8 ml min −1 and 0.5 ml fractions were collected for SDS–PAGE analysis. The column was calibrated using a calibration kit (Sigma). For the detection of the NIU complexes, 250 μl of a mixture containing 20 μM of the NI complex with equimolar amounts of ISCU (WT and cysteine mutants) was injected; for detection of the NIUF complexes, 200 μl of a mixture containing 100 μM of the NI complex with three equivalents of ISCU and five equivalents of the His-tagged version of FXN was injected. Synthesis of MalP 16 The maleimide-peptide compound MalP 16 comprises a maleimide moity linked to the 16-mer Leu-Val-Pro-Arg-Gly-Ser-Tyr-Lys-Gly-Thr-Ser-Lys-Leu-Asn-Tyr-Leu-NH 2 peptide. The peptide was elongated manually in a polyethylene syringe fitted with a polypropylene disc. Washing (3 × ) of the Rink amide resin with dichloromethane (DCM) and N,N -dimethylformamide (DMF) was followed by treatment with 20% piperidine/DMF (2 × 15 min) and washing (DCM, DMF, MeOH). Coupling conditions: 3 equivalents (eq.) of Fmoc-amino acid, 1-hydroxybenzotriazole and N,N ′-diisopropylcarbodiimide (minimum amount of DCM and a few drops of DMF, 90 min), followed by washing (DCM, DMF and MeOH). Incomplete couplings (Kaiser test) were repeated with 2 eq. of reagents. Removal of Fmoc groups: 20% piperidine/DMF (1 × 3 min+1 × 10 min), followed by washing (DMF, DCM). Activation of 3-maleimidopropanoic acid was carried out with the carbodiimide. Final deprotection conditions: 90:5:5 TFA:H 2 O:triisopropylsilane (2 × 1 h). Collected filtrate and DCM washings were concentrated under an N 2 stream and cold diethyl ether (10 volumes) was added to the resulting oil. The mixture was centrifuged (10 min, 5 °C, 4,800 r.p.m.) and decanted. This procedure was repeated three times. High-performance liquid chromatography (HPLC) purification: Phenomenex semipreparative Jupiter Proteo column (10 μm, 90 Å, 250 × 10 mm), A: 0.1% TFA in water, B: 0.1% TFA in acetonitrile, 3 ml min −1 , 280 nm, linear gradient from 25 to 50% of B. Fractions containing the pure peptide were pooled and lyophilized. Overall yield (from ultraviolet quantification, Tyr: 280 =1,480 M −1 cm −1 ): 22%. Analytical HPLC: Jupiter Proteo column (4 μm, 90 Å, 250 × 4.6 mm), A: 0.045% TFA in water, B: 0.036% TFA in acetonitrile, 1 ml min −1 , 280 nm, linear gradient from 20 to 40% of B in 30 min, t R =13.3 min. Matrix-assisted laser desorption/ionization-time-of-flight mass spectrometry (reflector, 2,5-dihydroxybenzoic acid+0.1% TFA, positive mode): m/z 1,946.4 [M+H] + , 1,968.4 [M+Na] + , 1,984.4 [M+K] + ; M calc. for C 89 H 140 N 24 O 25 1,945.0. Maleimide-peptide alkylation assay The MalP 16 was dissolved in purified water. All maleimide-peptide alkylation assays, unless indicated, were performed in buffer C using 25 μM NFS1–ISD11 and equimolar amounts of ISCU (WT and mutants) and/or FXN. For studies of persulfide formation, the reactions were initiated with L -cysteine (500 μM) and incubated at 25 °C. For studies of persulfide reduction, fully persulfurated NFS1 and ISCU were generated by incubating the NI complex in the presence of equimolar amounts of FXN or FXN and ISCU (NIUF complex) for 3 min and the NIU complex for 25 min at 25 °C with 500 μM L -cysteine to reach completion of the trans -persulfuration reaction. Excess L -cysteine was removed by desalting on micro-BioSpin6. Next the reduction reactions were initiated by adding the reductant and the complexes were incubated at 25 °C. Most experiments were performed with DTT (1 mM) as a reductant. Other reductants were also tested: GSH (1 mM), reduced FDX2 and Fe 2+ (see Supplementary Fig. 7 ). Reaction kinetics (formation and reduction) were monitored by sampling 10 μl of the reaction mixture at different time points, as indicated in the figures, and the reaction was stopped using either a 1.5-fold molar excess of MalP 16 relative to free thiols (protein cysteines, L -cysteine and possibly DTT) and SDS (2%) or TCA to a final concentration of 10%. For the TCA precipitation procedure, the reaction mixture was mixed with an equal volume of ice-cold TCA (20%) and the pellets were washed three times with ice-cold acetone. The protein pellets were resuspended in 10 μl buffer C containing 8 M urea and 10 mM MalP 16 . The reactions quenched by MalP 16 /SDS and TCA were incubated for 20 min at 30 °C, with constant shaking at 550 r.p.m. Half-reaction volumes were incubated with 1 μl of DTT at 100 mM for 20 min at 25 °C. Each reaction aliquot (7–8 μl) was analysed (500 ng of proteins) on 8 and 14% SDS–PAGE gels in non-reducing (without DTT) and reducing conditions (with DTT). TCA precipitation yielded essentially the same results as the MalP 16 /SDS quenching procedure, thus MalP 16 /SDS quenching was used on a day-to-day basis. Controls were used to determine the total number of cysteines available for alkylation by MalP 16 in NFS1, which contains seven cysteine residues, and ISCU, which contains four cysteine residues ( Supplementary Fig. 1a,c ). MalP 16 (2 eq.) relative to total sulfhydryl content were added to NFS1 (20 μM) or to a mixture of NFS1 (20 μM) and ISCU (20 μM) in buffer C, and the alkylation reaction was stopped after 30 s using the TCA procedure. Several other modifications engaging one or two cysteines could give rise to a false positive (non-alkylable cysteine residue), such as sulfenic, sulfinic or sulfonic acid, sulfenamide and disulfide bond, but this can be readily circumvented by analysing the proteins under non-reducing conditions where non-alkylable cysteines can be detected. Finally, the protein bands on SDS–PAGE were quantified using an Odyssey scanner (Li-Cor). The uncropped images of the gels used for the various figures are displayed in Supplementary Figs 11 and 12 . The data obtained for persulfide reduction by DTT and GSH were fitted assuming a bimolecular mechanism as demonstrated in multiple-turnover kinetics for NFS1 persulfide reduction (see Fig. 5c,d ) using equation (1) for second-order kinetic [42] , where S 0 is the initial concentration of reductant (DTT or GSH) and k R the bimolecular rate constant. The data of transfer were fitted assuming a monomolecular mechanism using equation (2) for first-order kinetic [42] . For studies as performed by Pandey et al . [12] , maleimide-peptide alkylation assays were performed in a final volume of 200 μl in buffer C using 50 nM of the NFS1–ISD11 complex with or without an equimolar amount of FXN. The reactions were initiated with 2 eq. of L -cysteine (100 nM) and were incubated for 15 min at 30 °C. The reactions were stopped using 50 eq. of MalP 16 relative to free thiols (cysteine from proteins and L -cysteine) and 2% SDS. The reaction mixtures were incubated for 20 min at 30 °C. Half-reaction volumes were incubated with 1 μl of 100 mM DTT for 20 min at 25 °C. The samples (85 μl) were concentrated using a SpeedVac apparatus to 20–25 μl. The samples were analysed on 8% SDS–PAGE gels in non-reducing (without DTT) and reducing conditions (with DTT). Cysteine desulfurase assays The amount of L -alanine generated during the reaction was determined using L -ADH, which generates 1 equivalent of NADH per L -alanine consumed (denoted ADH assay in the text). The reactions were performed in buffer C and initiated using L -cysteine at various concentrations as indicated in the figure legends and incubated at 25 °C. Samples (10, 20 or 30 μl) were withdrawn from the solution at various time points and the reaction was stopped using TCA precipitation (0.8% final). After 5 min of incubation on ice, the samples were centrifuged at 14,500 r.p.m. for 4 min at room temperature and NaOH at a final concentration of 70 mM was added to neutralize TCA. The reaction mixtures were then centrifuged again at 14,500 r.p.m. for 4 min at room temperature. Each sample was analysed in a final volume of 100 μl containing NAD + (6 mM) and L -alanine dehydrogenase (1 U) in 50 mM NaHCO 3 , pH 10. The kinetics of NADH formation was monitored at 340 nm during 20 min to reach completion. The curves were fitted assuming first-order kinetic [42] and the concentration of NADH corresponding to the total absorbance deviation at 340 nm was calculated using an extinction coefficient of 4,427 M −1 cm −1 (determined using L -alanine standard solutions). For determination of the stoichiometry of the complexes by dose–response experiments ( Supplementary Fig. 2f–h ), the reaction was performed with 20 μM of the NFS1–ISD11 complex and increasing amounts of FXN and/or ISCU in the presence of 0.5 mM L -cysteine and 1 mM DTT. Unless indicated, the other ADH assays were performed with 20 μM of the NFS1–ISD11 complex and equimolar amounts of ISCU (WT and mutants) and/or FXN. For determination of the kinetic parameters, steady-state conditions were cautiously controlled. Accordingly, the rate of alanine production reaches a steady-state (linear variation) after ~1 min for the NIUF complexes and 20 min for the NIU complex (corresponding to the time required for persulfuration of ISCU). Steady-state conditions were achieved in all cases by (1) monitoring L -alanine production at four different time points to ensure that the rates are actually linear and (2) selecting reaction times to ensure that no more than 30% of L -cysteine or DTT were consumed. For L -cysteine, we considered that three L -cysteine molecules are consumed for each L -alanine generated, as cysteine is also consumed by the reduction process. The initial velocities were determined from the linear regression using these four different time points. Fe-S cluster assembly Fe-S cluster assembly reactions were performed under anaerobic conditions in a glove box. Before introduction into the glove box, all the proteins were deoxygenated by flushing the head space with argon and the buffer by bubbling argon inside. The NSF1–ISD11 complex (50 μM) was mixed with equimolar amounts of ISCU with or without FXN in buffer C at 25 °C. Then, 4 eq. of Fe(NH 4 ) 2 (SO 4 ) 2 were added and the solutions were incubated for 2 min. The reactions were initiated using 30 eq. of L -cysteine (1.5 mM) with or without DTT (1.5 mM) and transferred to a septum-sealed cuvette. Ultraviolet–visible spectra between 200 and 800 nm were recorded every minute on a Cary 100 (Varian) spectrometer at 25 °C. Mass spectroscopy The samples analysed by ESI-Q/TOF were prepared using 40 μM of the NFS1–ISD11 complex with or without equimolar amounts of ISCU and/or FXN in buffer C at 25 °C. The reactions were initiated with 10 eq. of L -cysteine (400 μM) and incubated for 3 min at 25 °C. The samples were buffer exchanged in 50 mM NH 4 OAc, pH 7 buffer using micro-biospin6. Proteins were denatured for 5 min in 50% acetonitrile and 1% formic acid. Mass spectrometry measurements were performed with an electrospray Q/TOF mass spectrometer (Q/TOF Premier, Waters) equipped with the Nanomate device (Advion). Spectra were recorded with an estimated mass accuracy of ±1 Da. The HD_A_384 chip (5 μm i.d. nozzle chip, flow rate range 100−500 nl min −1 ) was calibrated before use. For ESI−MS measurements, the Q/TOF instrument was operated in RF quadrupole mode with the TOF data being collected between m/z 300 and 2,990 for whole proteins. Collision energy was set to 6 eV and argon was used as the collision gas. The Mass Lynx 4.1 software was used for acquisition and data processing. Deconvolution of multiply charged ions was performed by applying the MaxEnt1 algorithm. External calibration was performed with NaI clusters (2 μg μl −1 , isopropanol/H 2 O 50/50) in the acquisition m/z mass range. The samples analysed by Orbitrap-MS/MS were prepared in buffer C using 20 μM of the NIU and NIUF complexes. The reactions were performed with L -cysteine (400 μM) in a final volume of 20 μl for 1 min with the NIUF complex and 1 h with the NIU complex. Controls without L -cysteine were also analysed. The reactions were stopped by adding 5 μl of buffer C containing 20 mM of IAA and were incubated for 15 min at 30 °C in the dark. The alkylation reaction continues by adding 100 μl of buffer C containing 8 M urea and 50 mM IAA and incubate 1 h at 30 °C in the dark. Excess IAA was removed by TCA precipitation as described for the alkylation assay. The protein pellets were resuspended in 20 μl of buffer C containing 8 M urea. The samples were diluted 8 × in buffer C and incubated with trypsin (2% of total protein mass) for 2 h at 37 °C. Protein digests were analysed by nano-liquid chromatography (nano-LC) ESI tandem mass spectrometry (MS/MS). These were carried out on a U3000 Dionex nanoflow system connected to an LTQ Orbitrap XL mass spectrometer (Thermo Fisher Scientific) equipped with a nanoelectrospray source. The samples were run through a C18 nanocolumn (75 μm i.d. × 50 cm, PepMap100 C18, 3 μm, 100 Å; Dionex) after being injected onto a pre-concentration column with a flow rate of 20 μl min −1 of 0.1% TFA in water. Peptides were then loaded on the analytical column equilibrated with 0.1% of formic acid in water, and elution was carried out using a linear gradient from 2 to 60% of acetonitrile at a flow rate of 250 nl min −1 for 60 min. The mass spectrometer was operated in data-dependent mode to automatically switch between Orbitrap MS and MS/MS in the linear trap. Survey full scan MS spectra from 450 to 2,000 Da were acquired in the Orbitrap set to a resolution R =60,000 at m/z 400, after accumulation of 500,000 charges on the linear ion trap. The ions with the most intense signals (up to six, depending on signal intensity) were sequentially isolated for fragmentation and analysis of fragments in the linear ion trap using CID. Target ions already selected for MS/MS were dynamically excluded for 30 s. MS/MS raw files were individually processed through a Proteome Discoverer v1.3 (PD1.3) (Thermo Fisher Scientific, Les Ulis, France) workflow. Identification of proteins and the search for post-translational modifications were done using the MASCOT search engine v2.4. For identification, a tolerance of 5 p.p.m. was used for the mass of the precursors and 0.8 Da for the mass of the fragments. The estimation of the percentages of persulfuration of the peptides was performed by determination of the ratio of areas under the peaks of the chromatograms. The areas were obtained by extracting and integrating the mass intensity of each precursor identified. The percentages are reported as the ratio of persulfurated versus total amount of the corresponding peptide (persulfurated+unmodified) assuming that persulfuration does not modify the ionization properties of the peptide. HPLC analysis The products of the cysteine desulfurase reaction were analysed using HPLC. The reactions were performed in buffer C at 25 °C using 2 μM NFS1–ISD11 complex in a final volume of 300 μl. The reaction was initiated with a 750-fold excess of L -cysteine and was incubated for 1 h at 37 °C. The small molecules were separated from proteins using Amicon ultra (0.5 ml) with a cutoff of 10 kDa. The filtrate, containing the small molecules, was derivatized using the ACCQ-fluo reagent kit. The samples (5 μl) were injected at a flow rate of 1 ml min −1 , at 35 °C, on an AccQ-Tag column connected to an Alliance 2695 HPLC apparatus equipped with a fluo detector W2475. The separations were performed using a gradient as described by the manufacturer. Statistical analysis and software All the graphics from the figures, unless indicated, display one representative experiment. The kinetic parameters and s.e. reported in the tables were determined from at least three independent experiments. Prism 4.2 (GraphPad software) was used to fit the curves and generate the figures. ChemDraw Ultra 12.0 (CambridgeSoft) was used to draw the molecules. How to cite this article: Parent, A. et al . Mammalian frataxin directly enhances sulfur transfer of NFS1 persulfide to both ISCU and free thiols. Nat. Commun. 6:5686 doi: 10.1038/ncomms6686 (2015).